Cascaded logic gates in nanophotonic plasmon networks Optical computing has been pursued for decades as a potential strategy for advancing beyond the fundamental performance limitations of semiconductor-based electronic devices, but feasible on-chip integrated logic units and cascade devices have not been reported. Here we demonstrate that a plasmonic binary NOR gate, a 'universal logic gate', can be realized through cascaded OR and NOT gates in four-terminal plasmonic nanowire networks. This finding provides a path for the development of novel nanophotonic on-chip processor architectures for future optical computing technologies. Modern semiconductor-based electronics is rapidly approaching fundamental limits caused by interconnect delays and large heat generation. Photonic devices and circuits could potentially solve these problems, because photons have intrinsically higher information-carrying capacity and produce low heat loads [1] , [2] ; but, the goal of all-optical computing has remained elusive. Previous developments have centred on two routes towards optical logic gates: the first one based on linear optical effects, such as interferometry [3] , [4] , [5] , and the second one based on nonlinear processes, for example, tunable refractive indices or frequency mixing [6] , [7] , [8] . However, the diffraction limit of light has presented a fundamental obstacle for reducing the dimensions of optical logic components to the length scales of electronic devices in integrated circuits. During the past decade, it has been proposed that photonics based on surface plasmons, that is, quanta of collective electron oscillations strongly coupled to photons in metal nanostructures, constitute one of the most interesting avenues towards further scaling down of photonic devices [9] , [10] , [11] , [12] , [13] , [14] , [15] , [16] , [17] , [18] and simultaneous integration with solid-state electronics [19] , [20] , [21] . Indeed, plasmonics is now actively pursued as a core methodology for nanoscale optical interconnects [22] , [23] , [24] . We recently demonstrated a complete family of basic logic functions, that is, AND, OR and NOT gates, in simple photonic networks composed of interconnected silver nanowires25. The logic operations were realized by utilizing polarization and phase-dependent interference between plasmon beams propagating through the wire network. But more complex logic functions and functional photonic circuits rely on the possibility of cascading the basic gates. A particularly important step in this direction is the construction of the so-called universal gates, that is NAND and NOR gates, which can be combined to implement essentially any logic operation. Here we show that it is possible to cascade OR and NOT gates to realize a plasmonic inverse NOR gate in a four-terminal branched silver nanowire network. We use quantum dot (QD) near-field imaging to trace the plasmon wave packets through the branched network and to demonstrate precise control of optical interferences at the nanoscale. We believe that these observations and results may pave the way for the development of tomorrow's plasmon circuits for on-chip integrated optical computing. 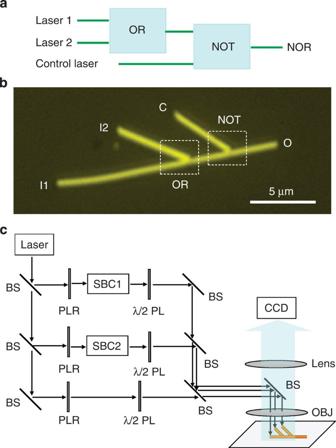Figure 1: Cascaded logic gates for NOR gate and the experimental setup. (a) Schematic illustration of logic gate NOR built by cascaded OR and NOT gates. (b) Optical image of the designed Ag NW structure. (c) Schematics of experimental setup. BS, beamsplitter; OBJ, objective; PLR, polarizer; SBC, Soleil-Babinet compensator; λ/2 PL, half-wave plate. Cascaded plasmonic OR and NOT gates for NOR gate Figure 1a illustrates the schematics of cascaded plasmonic OR and NOT gates for the universal logic gate NOR. It has recently been demonstrated that the interferences of two plasmon beams in single-branched Ag NW structure can function as OR or NOT gates [25] . Here we arranged Ag NWs ( Supplementary Fig. S1 ) with a micromanipulator to construct a four-terminal NW structure composed of a primary NW and two-branch NWs as shown in Figure 1b . The typical process for the construction of a NW network is shown in Supplementary Figure S2 for example. The first branch NW with the terminal marked as 'I2' and the first half-part of the primary NW with terminal marked as 'I1' form the first branched structure, which is designed to function as an OR gate. The second branch NW with the terminal marked as 'C' and the last-half part of the primary NW forms the second branched structure, which is designed to be a NOT gate. Figure 1: Cascaded logic gates for NOR gate and the experimental setup. ( a ) Schematic illustration of logic gate NOR built by cascaded OR and NOT gates. ( b ) Optical image of the designed Ag NW structure. ( c ) Schematics of experimental setup. BS, beamsplitter; OBJ, objective; PLR, polarizer; SBC, Soleil-Babinet compensator; λ/2 PL, half-wave plate. Full size image The propagating plasmons in the network can be launched through the excitation at the terminals marked as I1, I2 and C, or any combinations of them. It was known that the propagating plasmons in Ag NWs can be launched by laser excitation at the NW terminals or other discontinuities, such as nanoparticle-nanowire junctions [26] , [27] , [28] . In single-branched NW structures composed of a primary NW and a branch NW, the plasmons on the NW can also be excited by laser illumination at the branch tip [25] , [29] . If two plasmon beams are generated on the primary NW by excitation at the primary NW tip and the branch tip, these two beams will interfere on the NW and modulate the near field distribution and the output scattering intensity. Plasmonic OR or NOT gates can be obtained by tuning the intensity, phase and polarization of the incident lasers. With same mechanism, in cascade structures as in Figure 1b , the first branched Ag NW structure can function as OR gate by tuning the incident lasers at its input terminals, whereas the second branched structure functions as NOT gate to invert the output 'state' of the first structure by tuning the incident laser at its branch tip C. The optical setup is schematically shown in Figure 1c . A 633-nm laser is divided into three beams by beam splitters, and the polarization of each beam can be controlled by half-wave plates. Soleil-Babinet compensators are inserted into two of the beams, which can control the phase difference of these beams. These three beams were focused on the three input terminals of plasmonic NOR gate as shown in Figure 1b . If any two excitation beams are incident on two different terminals, the plasmons launched by these two laser beams will interfere in the branched NW structures. The output intensity will depend on the phase difference of these two laser beams [25] . By continuously changing the phase of one incident laser with a compensator, the intensity of the emitted light at the output end marked as 'O' will oscillate between the maximum value and the minimum value. 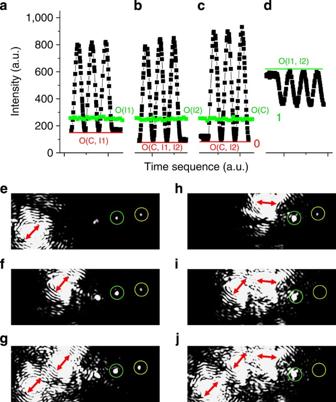Figure 2: Output intensity at the O end for different inputs versus the time sequence as the incident phases are changed. (a–d) The output intensity for the inputs from terminals (C, I1), (C, I1, I2), (C, I2) and (I1, I2). The red lines emphasize the output intensity for the NOR operation. The green line emphasizes the corresponding output intensity for (I1, I2). (e–g) The scattering images showing the OR operations. (h) The scattering image when only C was enabled. (i,j) The scattering images for the NOR operations, corresponding to a NOT function acting on (f,g). The red arrows show the incident laser polarization. The green and yellow circles mark the C-branch junction and the O terminal, respectively. Figure 2a shows the case for two inputs from the I1 and C terminals. The phase difference is controlled by tuning the compensator 1 in the light path for the I1 input. When the output intensity gets to the minimal value, further tuning of the compensator was stopped and the phase from I1 was fixed. A third laser beam is then applied to terminal I2. All three plasmon beams will interfere on the primary wire. By tuning the phase of the I2 input with another compensator, the output intensity will oscillate between a new minimum and maximum value as shown in Figure 2b . When the output intensity reached minimum, the I2 phase was fixed by stopping tuning of the corresponding compensator 2. At this time, the I1 beam was blocked so that only I2 and C interfere. It is found that the output is also the minimum to compare with other different interferences between I2 and C by changing the phase of I2 as shown in Figure 2c . That is to say, there is a particular given phase of I1 and I2 for which the outputs O(C, I1), O(C, I2), and O(C, I1, I2) are simultaneously minimized while the output O(I1, I2) is close to maximum as shown in Figure 2d . Figure 2: Output intensity at the O end for different inputs versus the time sequence as the incident phases are changed. ( a – d ) The output intensity for the inputs from terminals (C, I1), (C, I1, I2), (C, I2) and (I1, I2). The red lines emphasize the output intensity for the NOR operation. The green line emphasizes the corresponding output intensity for (I1, I2). ( e – g ) The scattering images showing the OR operations. ( h ) The scattering image when only C was enabled. ( i , j ) The scattering images for the NOR operations, corresponding to a NOT function acting on ( f , g ). The red arrows show the incident laser polarization. The green and yellow circles mark the C-branch junction and the O terminal, respectively. Full size image If we define a scattering intensity from the output terminal of >200 as the '1' or 'ON' state, for example, the value above the green dot lines (O(I1), O(I2), O(C)) in Figure 2a–c , and the intensity <200, for example, the red lines as '0' or 'OFF' state, then all of the two inputs interferences and the three inputs interferences result in '0' output for certain input phases. To illustrate the optical binary logic NOR gate, we treat terminal I1 and I2 as the input ends for the signals, and terminal C as the control end. For any input from either I1 or I2 only, the control C will invert it, that is, invert '0' to '1', or '1' to '0'. Hence, if we have input variables from (I1, I2): (0, 0), (1, 0), (0, 1), (1, 1), the output is 1, 0, 0, 0, respectively. That is the Boolean logic gate NOR, as shown in Table 1 . Table 1 Outputs of logic gates. Full size table To demonstrate that this plasmonic NOR gate is actually caused by cascading a plasmonic OR gate and a NOT gate, the scattering images for different inputs are shown in Figure 2e–j . Figure 2e–g clearly shows the outputs are ON when either or both I1 and I2 are ON, thus functioning as an OR gate. When control C is enabled, and I1 and I2 are disabled, as shown in Figure 2h , the output is ON, which means a NOT function. When this NOT function acts on the OR gate, then it will invert the output to be OFF, when either or both I1 and I2 are ON, as shown in Figure 2i,j . From Figure 2e–j , we firstly demonstrate OR gate, then let NOT gate function with C input enabled, and the overall effect is the NOR gate. Therefore, we have illustrated that the plasmonic NOR gate in this four-terminal structure designed here is composed of cascaded plasmonic OR and NOT gates. The outputs of different gates for each combination of the three input variables are shown in Table 1 . When the principle of cascaded plasmonic devices for NOR gate is understood, we can design different NWs network structures to realize NOR function based on the same principle. Supplementary Figure S3 shows another example of plasmonic NOR gate in a different four-terminal NW structure, that is, two-branch NWs locating at the different sides of the primary NW, but with the same logic function as shown in Table 1 as well. QD imaging reveals near-field distribution on NWs To understand the mechanism of cascaded plasmonic logic devices, we use QD fluorescence to image the electromagnetic (EM) near-field distribution of the propagating plasmons on metal NWs [25] . 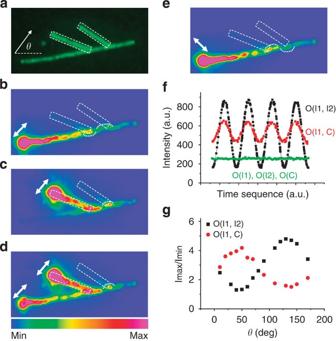Figure 3: Dependence of plasmon interference on incident polarizations. (a) QD fluorescence image by wide-field illumination. Dashed white lines show the outline of the branch NWs. (b–e) QD fluorescence images with excitation at different terminals with polarization indicated by the white arrows. (f) The output intensity at terminal O as a function of the phase difference between two laser beams. Green: the output intensity when only one input (I1, I2, or C) is applied. Black: the output intensity resulting from two incident beams (I1 and I2). Red: the output intensity resulting from two incident beams (I1 and C). The incident polarizations at I1 and I2 terminals used for this set of measurement corresponds to the polarizations shown in (e,c). The incident polarization at C terminal is the same as inFigure 2. (g) Interference depth of (I1, I2) and (I1, C) as a function of polarization angle θ of the input laser at the I1 terminal. The definition of θ is shown in (a). The polarizations of I2 and C are kept the same as those inFigure 2. Figure 3a shows the QD fluorescence image by a wide field excitation, which indicates an even distribution of QD coating on the NWs. The white dashed lines show the outline of the branch NWs. When the 633-nm laser was focused on only the I1 terminal with polarization of about 40°, as indicated by the white arrow in Figure 3b , corresponding to the scattering image shown in Figure 2e , the QD fluorescence image shows that the propagating plasmon energy has 'node-like' zigzag near-field distribution pattern. This pattern is caused by the superposition of different propagating plasmon modes induced by the incident laser at certain polarization, which modulates electric field distribution along the NW [25] , [30] , [31] . Figure 3: Dependence of plasmon interference on incident polarizations. ( a ) QD fluorescence image by wide-field illumination. Dashed white lines show the outline of the branch NWs. ( b – e ) QD fluorescence images with excitation at different terminals with polarization indicated by the white arrows. ( f ) The output intensity at terminal O as a function of the phase difference between two laser beams. Green: the output intensity when only one input (I1, I2, or C) is applied. Black: the output intensity resulting from two incident beams (I1 and I2). Red: the output intensity resulting from two incident beams (I1 and C). The incident polarizations at I1 and I2 terminals used for this set of measurement corresponds to the polarizations shown in ( e , c ). The incident polarization at C terminal is the same as in Figure 2 . ( g ) Interference depth of (I1, I2) and (I1, C) as a function of polarization angle θ of the input laser at the I1 terminal. The definition of θ is shown in ( a ). The polarizations of I2 and C are kept the same as those in Figure 2 . Full size image The white-dotted curved lines mark the outline of the EM field nodes at the two connection junctions between the branches and the main wire. It is interesting that the node position of zigzag pattern with strong EM near-field intensity overlapped with the position of the junction between the main wire and the C-branch wire. When the laser with the same polarization was focused on the terminal I2, the 'node-like' zigzag near-field pattern with strong EM near-field intensity again overlapped with the position of the connect junction of the C branch as shown in Figure 3c , which corresponds to the scattering image of Figure 2f . When these two lasers were focused on the I1 and I2 terminals simultaneously with the same phases as in Figure 2g , the zigzag pattern with strong EM near-field intensity also overlaps with the C-branch junction as shown in Figure 3d . In Figure 2e–g , we have demonstrated the function of plasmonic OR gate. As will be seen, the cascaded NOT gate will work when the zigzag pattern with the locally strongest EM field distribution overlaps with the C-branch junction. To make NOT gate work well, this kind of near-field distribution at the branch junction position is crucial to obtain sufficient interference between two plasmon beams (one in the main wire, and the other one in the branch) to make the output intensity sufficiently small as shown in Figure 2i,j , or the minimum values of (C, I1), (C, I2) and (C, I1, I2) in Figure 2a–c . Unlike the plasmonic NOT gate, significant interference is not required for the plasmonic OR gate. As shown in Figure 2d , the output scattering intensity O (I1, I2) can be somehow modulated by the interference between two plasmon beams I1 and I2 at different phases, but not as strongly as the interference between either or both of these two plasmon beams, and the plasmon beam from the C terminal is shown in O(C, I1), O(C, I2) and O(C, I1, I2) of Figure 2a–c , where the inverse logic function is needed to perform the NOR operation. If we check the zigzag pattern of EM near-field distribution shown in Figure 3b , the locally most intense part is located at the opposite side of the junction between the primary wire and the branch wire (I2). Evidently, strong interference requires that two beams should meet closely at the beginning, that is, the wave packet position with strong EM intensity should overlap with the connecting junction. Hence, the degree of such overlapping will determine how well the beams interfere. It should be noted that, although the junction of the C branch in Figure 3b–d is located at the stronger EM field position, it is deviated from the centre of the EM field packet in Figure 3b compared with Figure 3c,d . This may explain why the destructive interference for O(C, I1) is not as good as for O(C, I2) and O(C, I1, I2), that is, the lowest value of O(C, I1) is higher than lowest values of O(C, I2) and O(C, I1, I2). To further verify our point about the relation between how strong the interference is and EM field intensity distribution, the EM near-field distribution pattern in the main wire is varied by changing the I1 input polarization. For example, rotating the laser polarization for about 130°, as shown in Figure 3e , suddenly changes the zigzag EM near-field distribution pattern from that in the Figure 3b . In Figure 3e , the intense EM field packet of the zigzag pattern is completely moved away from the C-branch junction, while the I2 branch junction overlaps with an intense EM field packet. Comparing with Figure 2a , the interference between C and I1 becomes much less strong, as shown in Figure 3f (red curve), while the interference between I1 and I2 becomes much stronger (black curve) compared with Figure 2d . We define how well the plasmon beams interfere, or the interference depth, as the ratio of maximum and minimum scattering intensity (Imax/Imin), when the phase of two plasmon beams differs by π. Figure 3g shows this ratio versus the incident polarization angle at the terminal I1. For the strongest interference between C and I1, occurring when the EM wave packet overlaps with the C-branch junction for the incident polarization as in Figure 3b , the interference between I1 and I2 is the weakest in our device demonstrated here, and the vice versa. Hence, the interference depth can be tuned by shifting the zigzag EM wave packet on or off the branch junctions with different incident polarization on the primary wire. This clearly shows that the zigzag EM field pattern on the wire can indeed function as 'switch' to control the interference of two plasmon beams in the NW network. It should be noted that the reverse incident polarization dependence of interference depth for (I1, I2) and (I1, C) observed here just occasionally happens for this structure, but it is not a required condition to realize the NOR function. As the NOR function is relied on the NOT function to reverse the state at the C junction, there should be no relevancy to the interference depth of (I1, I2). In Supplementary Figure S4 , the different incident polarization dependence of interference depth for (I1, I2) and (I1, C) is observed, which shows almost the same polarization dependence. Hence, to realize NOR operation, the incident polarization in the primary NW at I1 is only required to guarantee the stronger interference at the C junction, that is, the plasmon wave packet overlapping largely with the C junction. This incident polarization is usually in a range of tens of degrees. We have demonstrated that cascaded plasmonic OR and NOT gates can be used to form a plasmonic NOR gate in a four-terminal nanowire network by multiple-beam plasmon interference. As cascading plasmonic devices are now possible, more complex functions can be realized by the precise design of complex plasmonic waveguide networks. NOR and NAND gates, the so-called universal logic gates, are the important elements of Boolean logics and are crucial to modern electronic circuits, because any Boolean logic gate can be constructed from a suitable network of NOR gates only, or NAND gates only. Similarly, plasmonic NOR gates demonstrated here could have key roles to constitute a logical formal system of Boolean logic in future optical computing. Moreover, plasmonic devices of the type discussed here can be further miniaturized and it is likely that improvement of the materials and wire interconnects will greatly reduce signal losses, thereby maintaining signal thresholds for the logic operations. This could allow for on-chip integration of a large number of cascaded subwavelength logic units for complex optical processing. Finally, our plasmonic structures allow for coherent control of optical quantum interferences and may therefore have a role in the development of future photonic quantum computation devices [32] , [33] , [34] . Synthesis of Ag NWs and the construction of NW structures The Ag NWs were synthesized by a wet chemical method as reported in the literature [35] . The products of the chemical reaction were washed with ethanol by centrifugation and redispersed in ethanol. The diameter of the Ag NWs is between 200 and 350 nm and the length is a few to tens of microns. Nanowires of such diameters have good elasticity and good toughness, which facilitate the manipulation of these NWs. A micromanipulator (MMO-202ND, Narishige) is used to manipulate the NWs and build the designed structures without having the NWs damaged. After the branched NW structure was built, an Al 2 O 3 layer of 30 nm was deposited by atomic layer deposition. Then, QDs with emission wavelength centred at 655 nm were spincoated onto the sample. Optical measurements The optical measurements were based on an Olympus BX51 microscope equipped with a piezo stage of high positioning accuracy and a CCD camera. The 633 nm laser was focused on the sample by a ×100 (NA 0.95) objective. The light from the sample was collected by the same objective and directed to the CCD camera to get the images. For the QD fluorescence imaging, a 633 nm long pass edge filter was used to block the laser. How to cite this article: Wei, H. et al . Cascaded logic gates in nanophotonic plasmon networks. Nat. Commun. 2:387 doi: 10.1038/ncomms1388 (2011).